Gas diffusion enhanced electrode with ultrathin superhydrophobic macropore structure for acidic CO2electroreduction 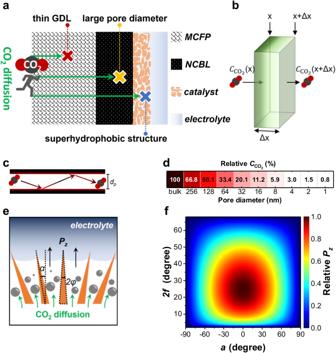Fig. 1: Modeling for CO2diffusion in a GDL. aIllustrations of CO2diffusion in the most common GDL. The thickness and pore diameter of the GDL, and the hydrophobicity of the catalyst together affect the CO2diffusion. (MCFP is macroporous carbon fiber paper and NCBL is nano-microporous carbon black layer).bCO2concentration (\({C}_{{{{\mbox{CO}}}}_{2}}\)) decreasing along diffusion distance (Δx).cKnudsen model for CO2diffusion through a pore with diameter (dp).dRelative\({C}_{{{{\mbox{CO}}}}_{2}}\)calculated towarddp.eIllustration of CO2diffusion on a needle-like architecture of the catalyst-electrolyte interface.Pzis Laplace pressure,2φis apex angle andαis tilt angle of the needle.f, RelativePzcalculated toward2φandα. Carbon dioxide (CO 2 ) electroreduction reaction (CO 2 RR) offers a promising strategy for the conversion of CO 2 into valuable chemicals and fuels. CO 2 RR in acidic electrolytes would have various advantages due to the suppression of carbonate formation. However, its reaction rate is severely limited by the slow CO 2 diffusion due to the absence of hydroxide that facilitates the CO 2 diffusion in an acidic environment. Here, we design an optimal architecture of a gas diffusion electrode (GDE) employing a copper-based ultrathin superhydrophobic macroporous layer, in which the CO 2 diffusion is highly enhanced. This GDE retains its applicability even under mechanical deformation conditions. The CO 2 RR in acidic electrolytes exhibits a Faradaic efficiency of 87% with a partial current density \(( {j}_{{{{\rm{C}}}}_{2+}})\) of −1.6 A cm −2 for multicarbon products (C 2+ ), and \( {j}_{{{{{{\rm{C}}}}}}_{2+}}\) of −0.34 A cm −2 when applying dilute 25% CO 2 . In a highly acidic environment, C 2+ formation occurs via a second order reaction which is controlled by both the catalyst and its hydroxide. Achieving effective utilization of carbon dioxide (CO 2 ) is of great significance for reducing the negative impacts of climate change and mitigating crisis caused by fossil fuel shortages [1] . Renewable electricity-driven CO 2 reduction reaction (CO 2 RR) to multicarbon (C 2+ ) products are highly demanded due to their high availability in various fields and current market price [2] . Over the past few years, a flow-type reactor has been used to investigate the CO 2 RR performance [3] , where gas reactants diffuse directly into catalyst-electrolyte interfaces through a gas diffusion layer (GDL), where CO 2 RR can occur at a high current density ( j ) [4] , [5] , [6] , [7] . Nevertheless, most reports have used strong alkaline electrolytes to ensure high C 2+ selectivity in CO 2 RR, which causes severe non-Faradaic consumption of CO 2 due to preferential carbonate formation under alkaline conditions (CO 2 + OH − → CO 3 2− ) and results in lower carbon utilization [8] , [9] . Moreover, the long-term accumulation of carbonate leads to flooding of the gas diffusion electrode (GDE), which thereby terminates the reaction (Supplementary Fig. 1 ). The operation of CO 2 RR under acidic conditions therefore offers entirely different strategy to overcome the challenges of conventional alkaline electrolyte systems [10] . In recent years, the development of highly selective catalysts that can effectively suppress the hydrogen evolution reaction (HER) in acidic environments has become a research hotspot. While some advanced catalysts have made progress in mitigating HER, they suffer from a significant reduction in the CO 2 RR rate compared to alkaline environments [11] , [12] . The primary reason for this matter is the absence of a hydroxide ion (OH − ) in an acidic environment, which causes insufficient adsorption of acidic CO 2 gas molecules and limited diffusion of CO 2 to the catalyst-electrolyte interface, resulting in the prevalence of undesired HER, particularly at high j [10] , [11] , [12] . To achieve high j , it is critical to overcome these inherent limitations in CO 2 RR under acidic conditions. One potential approach is to increase the CO 2 concentration at the catalyst-electrolyte interface by increasing the CO 2 flux in the gas diffusion layer (GDL), which could serve as a simple and effective strategy to improve CO 2 RR efficiency. Furthermore, hydroxide (OH)-derived Cu catalysts (OH-Cu) have been considered promising for achieving high selectivity towards C 2+ compounds due to the presence of OH in the catalyst structure [13] , [14] . The OH-rich nature of the catalysts can help to increase the pH of the catalytic layer, effectively suppressing HER in acidic environments. In addition, GDEs are generally composed of brittle and inflexible carbon materials [15] , making GDEs a non-recoverable consumable. In this study, we conducted a systematic evaluation of the factors influencing CO 2 diffusion in the GDL. Based on our findings, we designed an all-metal gas diffusion enhanced Cu electrode (Cu-GDL) using OH-Cu as a catalyst. This Cu-GDL demonstrated both mechanical flexibility and applicability, making it suitable for various practical applications. We systematically evaluated the CO 2 RR performance in an acidic environment by optimizing the electrolyte pH, catalyst amount, CO 2 flow rate, electrolyte type and CO 2 concentration. We achieved a high Faradaic efficiency of 87% ( \({{{{{\rm{FE}}}}}}_{{{{{{\rm{C}}}}}}_{2+}}\) ) with a partial current density ( \({j}_{{{{{{\rm{C}}}}}}_{2+}}\) ) of –1.6 A cm −2 for C 2+ products, and a \({j}_{{{{{{\rm{C}}}}}}_{2+}}\) of − 0.34 A cm −2 that meets industrial applications even with diluted 25% CO 2 . We discovered unique kinetics of CO 2 RR on Cu-GDL under acidic conditions: the first-order reaction at pH 6 and the second-order reaction at pH 1. Moreover, the CO produced in CO 2 RR could be further reduced to C 2+ at slow CO 2 flow rates, leading to an enhancement of the single-pass conversion efficiency (SPCE) to 42%, while simultaneously increasing \({{{{{\rm{FE}}}}}}_{{{{{{\rm{C}}}}}}_{2+}}\) to 87%. Modeling for CO 2 diffusion in a GDL We first verified requirements for achieving a favorable CO 2 diffusion efficiency (CO 2 DE) based on the architecture of the GDL, which is a hydrophobic porous electrode. CO 2 DE for a GDL is described by considering Fick’s second law, Knudsen self-diffusion models and surface hydrophobicity (Supplementary Figs. 2 - 4 , details in Methods). We found that three aspects are crucial to enhance CO 2 DE (Fig. 1a ): (1) Thin GDL; The CO 2 concentration ( \({C}_{{{{{{\rm{CO}}}}}}_{2}}\) ) is inversely proportional to the diffusion distance ( Δx ), and high \({C}_{{{{{{\rm{CO}}}}}}_{2}}\) is realized at a site with small Δx as shown in Fig. 1b . (2) Large pore diameter; Given the frequent collisions between CO 2 molecules and nano/micropore walls (Fig. 1c ) [16] , \({C}_{{{{{{\rm{CO}}}}}}_{2}}\) is halved when the porous diameter is smaller than 128 nm, followed by a severe \({C}_{{{{{{\rm{CO}}}}}}_{2}}\) -limiting behavior with decreasing pore diameter (Fig. 1d , Supplementary Fig. 3 ). (3) Superhydrophobic structure; Considering that CO 2 diffusion coefficient in the gas phase is approximately four orders of magnitude higher than that in the liquid phase [17] , [18] , a hydrophobic interface formed between the catalyst surface and an electrolyte is an ideal space for the CO 2 diffusion. The positive Laplace pressure ( P z ) of a gas phase at an interface between liquid and nano/microscale texture is a measure for emergence of hydrophobicity (Supplementary Fig. 4 ) [19] . Thus, CO 2 can rapidly diffuse on catalyst-electrolyte interfaces characterized with a positive P z (Fig. 1e ). According to the Laplace equation, P z always shows a positive value when the tilt angle is −90° < α < +90° and the apex angle is 0° < 2 φ < 66°, and the maximum P z value can be achieved at α = 0° and 2 φ = 22° (Fig. 1f ). This assessment of GDL architectures led us to design a GDE with a thinner, macroporous diameter, as well as vertical and needle-like surface structures to facilitate CO 2 diffusion. Fig. 1: Modeling for CO 2 diffusion in a GDL. a Illustrations of CO 2 diffusion in the most common GDL. The thickness and pore diameter of the GDL, and the hydrophobicity of the catalyst together affect the CO 2 diffusion. (MCFP is macroporous carbon fiber paper and NCBL is nano-microporous carbon black layer). b CO 2 concentration ( \({C}_{{{{\mbox{CO}}}}_{2}}\) ) decreasing along diffusion distance ( Δx ). c Knudsen model for CO 2 diffusion through a pore with diameter ( d p ). d Relative \({C}_{{{{\mbox{CO}}}}_{2}}\) calculated toward d p . e Illustration of CO 2 diffusion on a needle-like architecture of the catalyst-electrolyte interface. P z is Laplace pressure, 2φ is apex angle and α is tilt angle of the needle. f , Relative P z calculated toward 2φ and α . Full size image Structural and compositional features of Cu-GDL GDEs are commonly prepared using nanoparticulate electrocatalysts and binders on GDL substrates [20] , but they do not meet the above requirements. In contrast, a porous Cu electrode, prepared by an in situ electrooxidation of a porous Cu foil, is sufficiently thin and has large pores, with its surface covered by special nanostructures. However, achieving vertical and needle-like structures with characteristic apex and tilt angles requires precise control of the incorporation rates of Cu 2+ and OH − on the Cu foil surface. By optimizing the synthetic conditions, we found that the balance between electrolyte concentration (KOH) and j for the electrooxidation of the Cu foil surface is the most important factor to construct favorable nanostructures (see Methods and Supplementary Figs. 5 – 7 for more details). The reaction temperature (0 °C) is also critical factor for achieving the vertical and needle-like structure with characteristic apex and tilt angles (see Methods and Supplementary Figs. 8 and 9 for more details). However, the as-prepared porous Cu easily penetrates the aqueous solution due to its large pore structure, which is unsuitable for use as a GDE in a flow cell. Therefore, we imparted water-barrier properties on the porous Cu surface by coating with 1-octadecanethiol, resulting in Cu-GDL [21] . A schematic diagram of Cu-GDL with enhanced CO 2 diffusion in CO 2 RR is shown in Fig. 2a . A scanning electron microscopy (SEM) image of Cu-GDL confirmed that the macroporous foil structure remains intact (Fig. 2b and Supplementary Fig. 10 ) and that nanoneedles are grown highly densely (Fig. 2b, c ). A cross-sectional SEM image of Cu-GDL confirmed the ultrathin structure of ~100 μm (Fig. 2d ), which is ~0.4 times thicker than a commercial carbon GDL (Supplementary Fig. 2 ). Energy dispersive X-ray (EDX) mapping analysis revealed that small amount (0.11 wt%) of S element of alkanethiol is uniformly distributed on the surface of Cu nanoneedle (Fig. 2e , Supplementary Fig. 11 ). Transmission electron microscopy (TEM) of Cu-GDL revealed that a Cu nanoneedle was coated with a layer of 1-octadecanethiol with a thickness of ~2.5 nm (Fig. 2 f and g), which corresponds to the chain length of 1-octadecanethiol between the surface-bound S and the terminal C [21] . It should be noted that X-ray photoelectron spectroscopy (XPS) for Cu 2 p revealed that the Cu nanoneedle coated with a layer of 1-octadecanethiol does not show any effect on the oxidation state of Cu (Supplementary Fig. 12 ). In addition, attenuated total reflectance Fourier transform infrared (ATR-FTIR) spectroscopy (Supplementary Fig. 13 ), XPS for S 2 p (Supplementary Fig. 14 ), and microscopic observations (Supplementary Fig. 15 ) further confirmed the existence of 1-octadecanethiol on Cu-GDL and its roles. The perpendicularly grown needle-like nanostructures on the surface were observed by SEM (Fig. 2d ). Such high-density nanoneedle structures could multiply the hydrophobicity according to the P z (see Eq. ( 4 )). The apex angle was determined to be in the range of 18–25° (Supplementary Fig. 16 ), which is very close to the perfect value of 22° suggested by our calculation of relative P z versus apex angles (Fig. 1f ). A contact angle (CA) measurement showed that Cu-GDL has superhydrophobicity characterized with a CA of 158.5° (Fig. 2c ). In contrast, an alkanethiol-modified original Cu foil exhibited normal hydrophobicity with a CA of 123.3°, which clearly indicates that superhydrophobicity of Cu-GDL originates from its surface structure and not only from the coating with the thiol layer (Supplementary Fig. 17 ). In addition, the nanostructures appear to be able to minimize the size of bubbles to enhance their desorption [22] , [23] , which is critical in terms of energy efficiency. Slow bubble removal from the electrodes is known to cause energy losses of up to 20% [24] , and therefore bubbles must be efficiently removed from GDL. It should be noted that our Cu-GDL retained its superhydrophobicity even after being severely bent (Fig. 2h ) and twisted (Fig. 2i ). Such a durable and flexible superhydrophobic GDL may contributes to the industrialization of CO 2 electroreduction. Fig. 2: Structural and compositional features of Cu-GDL. a Illustration of Cu-GDL applied in CO 2 RR. b , c SEM images for b macropores (the inset of b is the macroporous channel) and for c high-density nanoneedles exhibiting a large contact angle (CA). d Cross-sectional SEM images to confirm ultrathin electrode thickness and vertically grown nanoneedles. e Elemental distribution. (red is Cu, green is S). f , g TEM images covered with ~2.5 nm 1-octadecylthiol single layer as a hydrophobic layer. h Bending resistance test. i , Twisting resistance test. Full size image Surface states of Cu-GDL X-ray diffraction (XRD) patterns confirmed that the major component of Cu-GDL is metallic Cu (Fig. 3a ). Interestingly, ex situ Raman spectroscopy revealed similar Raman signals around 431, 528, and 623 cm −1 for both Cu-GDL and Cu(OH) 2 (Supplementary Fig. 18 ) [25] . However, no peaks related to Cu 2+ were observed in the XPS for Cu 2 p (Supplementary Fig. 12 ). Furthermore, XPS for O 1 s revealed the presence of OH on the surface of Cu-GDL (Supplementary Fig. 19 ) [14] . These findings indicate that the composition of Cu-GDL consists mainly of metallic Cu covered with OH. To investigate the effect of acidic electrolyte on the electrode composition in CO 2 RR, in situ Raman spectroscopy was conducted at a potential ( E ) of −1.5 V vs SHE using electrolytes of pH 6 and pH 1, which suggested that OH is stably present on the Cu-GDL even in a highly acidic solution under the potential (Fig. 3b ). Given various influential factors such as current density, diffusion layer thickness, bulk electrolyte composition, and other factors, the determination of a pH just above the electrode surface, “intrinsic pH”, during CO 2 RR appears to be challenging [26] . To address this, we applied an electrochemical approach based on the onset potential for the oxidation of Cu 0 to Cu 1 , and the intrinsic pH on Cu-GDL was calculated from the onset potential observed on a pristine Cu foil as reference using Nernst equation (see Methods and Supplementary Fig. 20 for details). In this experiment, we used a slow scan rate of 10 mV s −1 at low j in the range of μA cm −2 , in an inert and near-neutral 0.1 M Ar-saturated KHCO 3 electrolyte. The test revealed that the catalyst surface has a pH of 10.9 (Fig. 3c ), suggesting the alkaline nature of the Cu-GDL surface, which would reduce local H + concentrations, and thereby suppress HER during CO 2 RR. Fig. 3: Surface states of Cu-GDL. a XRD pattern of Cu-GDL. b In situ Raman spectroscopy for Cu-GDL at pH 6 and pH 1 with E of − 1.5 V vs. SHE (Cu foil used as reference baseline, yellow stars mark bands associated with OH). c Evaluation of surface pH on Cu in 0.1 M Ar-saturated KHCO 3 . A yellow dashed curve represents a fitted line for the HER current. The onset oxidation potential of a Cu foil is 0.45 V (vs. RHE), and porous Cu is 0.35 V (vs. RHE). The pH difference (ΔpH) between a Cu foil and porous Cu is 1.7. Full size image CO 2 RR performance of Cu-GDL and underlying mechanisms The CO 2 RR performance was evaluated at j ranging from −0.3 to −1.8 A cm −2 by using acidic electrolytes. High \({{{{{\rm{FE}}}}}}_{{{{{{\rm{C}}}}}}_{2+}}\) of 87% and low Faradaic efficiency for HER less than 4% were achieved at both pH 6 and pH 1 (Fig. 4a , Supplementary Fig. 21 ). The Cu-GDL retains its original morphology after CO 2 RR operation (Supplementary Fig. 22 ). Fig. 4: CO 2 RR performance of Cu-GDL and underlying mechanisms. a FE for the production of C 2+ and H 2 , and potential (E vs. RHE, right) as functions of j (pH 6 is blue, pH 1 is red). b rf (left) and rf 2 (right) as functions of \({{{{{{\rm{FR}}}}}}}_{{C}_{2+}}\) . Inset shows the SEM images of Cu-GDL having corresponding rf (error bars = 2 μm). c Illustration of a function of OH species on Cu-GDL during CO 2 RR in acidic media. d SPCE, e CO selectivity and f C 2+ selectivity as a function of CO 2 flow rate at an applied j of −0.5 A cm −2 using electrolytes with pH = 6 (pH 6) and pH = 1 (pH 1) and CO 2 saturated electrolytes with pH = 3.8 (pH 6_CO 2 ) and pH = 0.9 (pH 1_CO 2 ). g Illustration of secondary CO conversion during CO 2 RR at a slow CO 2 flow rate. h Carbon utilization percentage at CO 2 flow rate of 3.5 sccm and an applied j of −0.5 A cm −2 at varying electrolyte. i \({j}_{{{{\mbox{C}}}}_{2+}}\) as a function of \({C}_{{{{\mbox{CO}}}}_{2}}\) (diluted gas is N 2 ). j Comparison of \({{{\mbox{FE}}}}_{{{{\mbox{C}}}}_{2+}}\) , \({{{\mbox{FE}}}}_{{{{\mbox{H}}}}_{2}}\) , \({j}_{{{{\mbox{C}}}}_{2+}}\) , SPCE and pH of bulk electrolyte on Cu-GDL with those on the state-of-the-art CO 2 RR in acidic media. a , b , d , e , f , i , error bars indicate s.d. ( n = 3 replicates). Full size image We first optimized the catalyst amount by changing the reaction time for the electrooxidation of a Cu foil. The original Cu foil coated with 1-octadecanethiol hardly participated in CO 2 RR, and both the \({j}_{{{{{{\rm{C}}}}}}_{2+}}\) and the formation rate of C 2+ ( \({{{{{\rm{FR}}}}}}_{{{{{{\rm{C}}}}}}_{2+}}\) ) tended to increase with increasing the electrooxidation time (Supplementary Figs. 23 and 24 ). To understand the relationship between the catalytically active surface area and \({{{{{\rm{FR}}}}}}_{{{{{{\rm{C}}}}}}_{2+}}\) , we further evaluated the roughness factors (rf) of each electrode by analyzing electrochemical surface area (ECSA), which reflects the number of catalytic sites (Supplementary Fig. 25 ). The SEM images of the electrodes corresponding to the rf are shown in Fig. 4b . Considering that the high selectivity of Cu-GDL towards C 2+ is accompanied by minimal HER, we established the relationship between the \({{{{{\rm{FR}}}}}}_{{{{{{\rm{C}}}}}}_{2+}}\) and rf (Supplementary Fig. 26 ). Interestingly, there was a good linear correlation between \({{{{{\rm{FR}}}}}}_{{{{{{\rm{C}}}}}}_{2+}}\) and rf at pH 6, whereas \({{{{{\rm{FR}}}}}}_{{{{{{\rm{C}}}}}}_{2+}}\) showed nonlinear behavior at pH 1 (Fig. 4b , Supplementary Fig. 26 ). Since the as-prepared Cu-GDL has an OH-rich surface, which reduces the local H + concentration, we reasoned that not only the active surface area but also the amount of OH present on the catalyst simultaneously determines the \({{{{{\rm{FR}}}}}}_{{{{{{\rm{C}}}}}}_{2+}}\) at pH 1 as described in Fig. 4c . We then attempted tried to analyze the relationship between \({{{{{\rm{FR}}}}}}_{{{{{{\rm{C}}}}}}_{2+}}\) and the quadratic roughness factor (rf 2 ). Surprisingly, \({{{{{\rm{FR}}}}}}_{{{{{{\rm{C}}}}}}_{2+}}\) showed a very good linear correlation with rf 2 at pH 1 (Fig. 4b ). Although the kinetics of CO 2 RR may involve various influencing factors, we made a predictive investigation of CO 2 RR kinetics in an acidic environment by precisely controlling the variables and found that CO 2 RR on Cu-GDL at pH 6 is a first-order reaction depending on the number of catalytic sites, whereas CO 2 RR at pH 1 can be described as a second-order reaction which is determined by the number of catalytic sites and the amount of OH. In this regard, we further characterized OH concentration on each electrode (Supplementary Fig. 27 ) and determined the rate constants of CO 2 RR ( k ) at pH 6 and pH 1 to be 4.20 × 10 2 h −1 and 2.45 × 10 1 μmol −1 cm 2 h −1 , respectively (Supplementary Fig. 28 ) [27] . Next, we evaluated the carbon utilization in CO 2 RR at −0.5 A cm −2 with CO 2 flow rate ranging from 10 to 3 sccm. Considering that the possibility to improve the recovery of CO 3 2− to CO 2 during CO 2 RR, which has been considered as a key to enhance CO 2 utilization [12] , we additionally employed two sets of electrolytes; CO 2 -saturated electrolytes with pH 6 and pH 1, namely pH 6_CO 2 and pH 1_CO 2 . The carbon utilization tests suggested that both SPCE and conversion efficiency for C 2+ ( \({{{{{\rm{CE}}}}}}_{{{{{{\rm{C}}}}}}_{2+}}\) ) gradually increase as the CO 2 flow rate decreases (Fig. 4d , Supplementary Fig. 29 ), and the corresponding \({{{{{\rm{FE}}}}}}_{{{{{{\rm{C}}}}}}_{2+}}\) are shown in Supplementary Fig. 30 and 31 . At a CO 2 flow rate of 3.5 sccm, it simultaneously exhibited the optimal SPCE of 42% and the optimal \({{{{{\rm{FE}}}}}}_{{{{{{{\rm{C}}}}}}}_{2+}}\) of 87% (Fig. 4d , Supplementary Fig. 31 ). However, when the flow rate was reduced to 3 sccm, the SPCE did not increase further beyond 42% as the CO 2 flow rate decreased (Fig. 4d ). On the contrary, the HER increased to 19–26% (Supplementary Fig. 32 ). This result suggests that CO 2 supply via recovery from the CO 3 2− dissolving electrolyte is not effective for improving SPCE, even when we use the CO 3 2− -rich and CO 2 saturated electrolytes. We then propose that this phenomenon can be attributed to the fact that CO 2 recovered from CO 3 2− tends to remain in the liquid phase. The CO 2 diffusion efficiency in the liquid phase is greatly reduced compared to the gaseous phase [17] , [18] . The encouraging point is that, when considering the formation of CO 3 2− during CO 2 RR, our SPCE results remain above 40% for both pH 6 and pH 1 conditions, exceeding the theoretically maximum achievable SPCE. The calculation results are summarized in Supplementary Tables 1 and 2 and used for comparison (see Methods). Further analysis of the product selectivity showed that the selectivity of CO decreases with decreasing of CO 2 flow rate (Fig. 4e ), resulting in a continuous increase of the selectivity of C 2+ (Fig. 4f ). This result leads us to conclude that a part of the theoretical maximum SPCE originates from the CO secondary conversion of as described in Fig. 4g . CO secondary conversion refers to the fact that the low CO 2 flow rate results in a prolonged residence time of CO, derived from CO 2 conversion, on the catalyst surface. Consequently, CO is further reduced, leading to the C 2+ formation. Importantly, an enhancement in SPCE is observed due to the absence of side reactions involving CO 3 2− formation during the carbon monoxide reduction (CORR) process [28] . 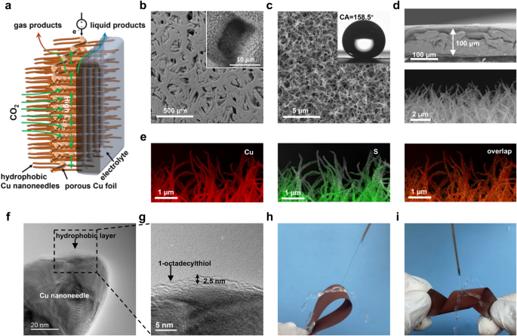Fig. 2: Structural and compositional features of Cu-GDL. aIllustration of Cu-GDL applied in CO2RR.b,cSEM images forbmacropores (the inset ofbis the macroporous channel) and forchigh-density nanoneedles exhibiting a large contact angle (CA).dCross-sectional SEM images to confirm ultrathin electrode thickness and vertically grown nanoneedles.eElemental distribution. (red is Cu, green is S).f,gTEM images covered with ~2.5 nm 1-octadecylthiol single layer as a hydrophobic layer.hBending resistance test.i, Twisting resistance test. Calculated carbon utilizations in CO 2 RR at a CO 2 flow rate of 3.5 sccm are summarized in Supplementary Table 2 , which shows that 30.3–31.7% of the carbon products come from CO 2 conversion, 7.6–9.5% from CO conversion, and 59.0–60.8% of the CO 2 is used for CO 3 2− formation (Fig. 4h ). In view of the enhanced CO 2 diffusion properties of Cu-GDL, we further evaluated the CO 2 RR performance in the presence of N 2 impurity gas (Supplementary Fig. 33 ). The CO 2 RR performance indicated that the influence of \({C}_{{{{{{\rm{CO}}}}}}_{2}}\) on the \({{{{{\rm{FE}}}}}}_{{{{{{\rm{C}}}}}}_{2+}}\) is limited, but remarkable on the \({j}_{{{{{{\rm{C}}}}}}_{2+}}\) (Fig. 4i , Supplementary Fig. 34 ). The \({j}_{{{{{{\rm{C}}}}}}_{2+}}\) for diluted 25% CO 2 gas reached −430 and −280 mA cm −2 at pH 6 and pH 1, respectively (Fig. 4i ). Even at such low \({C}_{{{{{{\rm{CO}}}}}}_{2}}\) , the productivity levels are still in a regime of interest with respect to industrial application [29] . The CO 2 RR performance of Cu-GDL was compared with those of state-of-art CO 2 RR in acidic media as shown in Fig. 4j [10] , [11] , [12] . In addition, in previous systems, the continuous accumulation of CO 3 2− during CO 2 RR required procedures such as stopping the reaction and replacing the electrolyte to maintain CO 2 RR activity [4] , [30] , [31] . However, these procedures significantly increased the operating costs associated with CO 2 RR. To address this issue, we designed an automatic electrolyte recovery system (Supplementary Fig. 35 ) that can maintain a CO 3 2− free electrolyte during the CO 2 RR operation by introducing a small amount of HCl to decompose carbonates: CO 3 2− + H + → CO 2 ↑ . 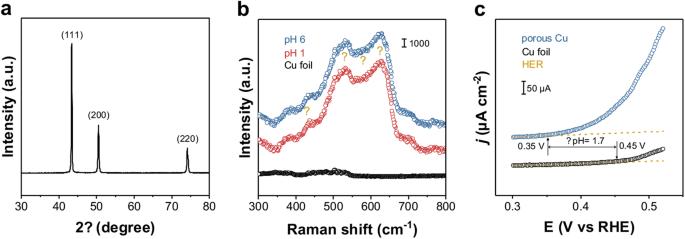Fig. 3: Surface states of Cu-GDL. aXRD pattern of Cu-GDL.bIn situ Raman spectroscopy for Cu-GDL at pH 6 and pH 1 with E of − 1.5 V vs. SHE (Cu foil used as reference baseline, yellow stars mark bands associated with OH).cEvaluation of surface pH on Cu in 0.1 M Ar-saturated KHCO3. A yellow dashed curve represents a fitted line for the HER current. The onset oxidation potential of a Cu foil is 0.45 V (vs. RHE), and porous Cu is 0.35 V (vs. RHE). The pH difference (ΔpH) between a Cu foil and porous Cu is 1.7. 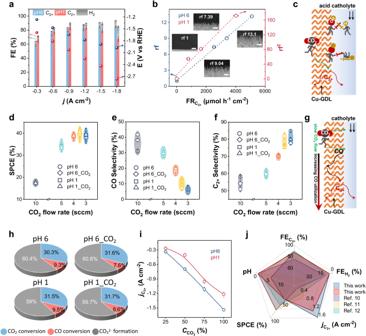Fig. 4: CO2RR performance of Cu-GDL and underlying mechanisms. aFE for the production of C2+and H2, and potential (E vs. RHE, right) as functions ofj(pH 6 is blue, pH 1 is red).brf (left) and rf2(right) as functions of\({{{{{{\rm{FR}}}}}}}_{{C}_{2+}}\). Inset shows the SEM images of Cu-GDL having corresponding rf (error bars = 2 μm).cIllustration of a function of OH species on Cu-GDL during CO2RR in acidic media.dSPCE,eCO selectivity andfC2+selectivity as a function of CO2flow rate at an appliedjof −0.5 A cm−2using electrolytes with pH = 6 (pH 6) and pH = 1 (pH 1) and CO2saturated electrolytes with pH = 3.8 (pH 6_CO2) and pH = 0.9 (pH 1_CO2).gIllustration of secondary CO conversion during CO2RR at a slow CO2flow rate.hCarbon utilization percentage at CO2flow rate of 3.5 sccm and an appliedjof −0.5 A cm−2at varying electrolyte.i\({j}_{{{{\mbox{C}}}}_{2+}}\)as a function of\({C}_{{{{\mbox{CO}}}}_{2}}\)(diluted gas is N2).jComparison of\({{{\mbox{FE}}}}_{{{{\mbox{C}}}}_{2+}}\),\({{{\mbox{FE}}}}_{{{{\mbox{H}}}}_{2}}\),\({j}_{{{{\mbox{C}}}}_{2+}}\), SPCE and pH of bulk electrolyte on Cu-GDL with those on the state-of-the-art CO2RR in acidic media.a,b,d,e,f,i, error bars indicate s.d. (n= 3 replicates). By implementing the electrolyte renewal system, we were able to achieve continuous operation of CO 2 RR at a pH ≈ 1 for more than 10 h with an applied j of −600 mA cm −2 (Supplementary Fig. 36 ), and for more than 30 h with an applied j of −200 mA cm −2 (Supplementary Fig. 37 ). In the future, the development of a more stable hydrophobic layer that surpasses the stability of thiols holds promise for further improving the long-term stability of CO 2 RR at high j . We first validated CO 2 DE of the conventional GDL and found that CO 2 DE can be improved by optimizing thickness, pore size, and hydrophobicity of GDL. Based on the analysis results, we designed a novel Cu-GDL exhibiting ultrathin, macroporous and superhydrophobic properties. It should be noted that Cu-GDL maintained its applicability even under severe bent and twisted states. By employing Cu-GDL, we achieved a \({{{{{\rm{FE}}}}}}_{{{{{{\rm{C}}}}}}_{2+}}\) of 87% at \({j}_{{{{{{\rm{C}}}}}}_{2+}}\) of −1.6 A cm −2 under acidic conditions and discovered that CO 2 RR on Cu-GDL is characterized as a first-order reaction at pH 6 and a second-order reaction at pH 1. We proposed the secondary CO conversion mechanism for the enhancement of SPCE in CO 2 RR. Furthermore, we achieved a \({j}_{{{{{{\rm{C}}}}}}_{2+}}\) of −0.34 A cm −2 even using diluted 25% CO 2 . Overall, understanding CO 2 RR systems on the enhanced gas diffusion electrode implemented in this work would accelerate the development of CO 2 RR technology. In the future, it would be useful to further investigate the influence of the local environment in the gas diffusion electrode using advanced in-situ detection methods. Modeling of CO 2 diffusion The CO 2 diffusion was assessed by assuming the architecture of GDE, which is hydrophobic porous electrodes [32] . Generally, the gas concentration change due to diffusion is predicted by Fick’s second law, which is determined by the following equation: 
    ∂C_CO_2/∂t=D∂^2C_CO_2/∂x^2
 (1) where \({C}_{{{{{{\rm{CO}}}}}}_{2}}\) is the concentration of CO 2 , t is time, D is the diffusion coefficient, x is crosswise position of the GDE. When \({C}_{{{{{{\rm{CO}}}}}}_{2}}\) is in a steady state, i.e. \({C}_{{{{{{\rm{CO}}}}}}_{2}}\) does not change with t , 
    ∂C_CO_2/∂t=0
 (2) Because a macropore structure does not limit CO 2 diffusion, \({C}_{{{{{{\rm{CO}}}}}}_{2}}\) in the macroprous carbon fiber paper (MCFP, Supplementary Fig. 2 ) having a constant D shows a linear dependence on x as shown in Fig. 1b and, therefore, the Fick’s second law suggests that CO 2 diffusion efficiency can be improved by thinning GDE. A nano-microporous carbon black layer (NCBL) is made up of nanoscale carbon black particles that forms a nano-microporous layer (Supplementary Fig. 2 ), and the pore sizes are further reduced when catalyst coating is applied [5] . In light of frequent collisions between CO 2 molecules and nano-micropore walls, as illustrated in Fig. 1c . The diffusion coefficient ( D ) in the nano-micropore domain is determined by Knudsen diffusivity [16] , which is described as follows: 
    D=(1/D_b+3/√(8RT/πM)d_p)^-1
 (3) where D b is the bulk diffusion coefficient of CO 2 (1.6 × 10 −5 m 2 s −1 ) [5] , R is the gas constant, T is temperature, M is molecular mass of CO 2 , d p is an average diameter of the nano-micropore. We calculated D based on Eq. ( 3 ) and suggested that \({C}_{{{{{{\rm{CO}}}}}}_{2}}\) is halved when d p becomes smaller than 128 nm, which probably causes severe CO 2 concentration-limiting behavior (Fig. 1d , Supplementary Fig. 3 ). As D values are approximately four orders of magnitude higher than those in the liquid phase [17] , [18] , preparing a superhydrophobic catalyst-electrolyte interface can prevent decay of the CO 2 diffusion rate. Nature often exhibits a superhydrophobic surface formed on its nano-microtextured structure [33] , such as lotus [34] , rice leaves [35] , water striders’ legs [36] and moth eyes [37] . A superhydrophobic surface shows a positive Laplace pressure ( P z ) from the gas present in a nano-microscale texture [19] . The P z can be expressed by using the following equation [30] : 
    P_z 	=2γ√(πΩf sinφ)[sin(θ_0-π/2-φ+α)+ sin(θ_0-π/2-φ -α)]/2
     	=γ√(πΩf sinφ) cosα sin(θ_0-π/2-φ)
 (4) where γ is the surface tension of the liquid, Ω is the density of the nano-microscale texture, f is the adhesion fraction of the liquid–solid interface, φ is half-angle of the apex, α is the tilt angle of the needle (Fig. 1e , Supplementary Fig. 4 ), and θ 0 is the static contact angle (123.3°), which obtained on surface of a porous Cu foil modified with 1-octadecanethiol (Supplementary Fig. 17 ). When the tilt angle is −90° < α < +90° and the apex angle is 0° < 2 φ < 66°, P z always shows a positive value (Fig. 1f ). Our calculations indicate the maximum P z value can be achieved at α = 0° and 2 φ = 22° (Fig. 1f ), which indicates that the vertical and needle-like structure reveals the marked hydrophobicity on its surface. Electrode preparation and optimization The preparation of GDE is based on the optimization of a previously reported in situ electrooxidation method [14] . A porous Cu foil was first washed with HCl (36%, Wako) for 1 min, followed immediately by ultrasonic cleaning with acetone (99.5%, Wako), ethanol (99.5%, Wako), and deionized water (18.2 MΩ cm −1 ) for 5 min to remove surface impurities. Based on the principle of in situ electrooxidation, the anode reaction can be described as follows: 
    [        Cu→Cu^2++e^-; OH^-+Cu^2+→Cu(OH)_2 ]
 (5) Upon examining the reaction formula, it becomes evident that the relative concentrations of OH – and Cu 2+ play a crucial role in facilitating the efficient occurrence of the electrooxidation process. Consequently, we conducted several optimizations to ensure favorable conditions. These included adjusting the KOH concentration in the electrolyte (which controls the OH – concentration, as shown in Supplementary Figs. 5 and 6 ), the electrooxidation current density (which controls the Cu 2+ concentration, as shown in Supplementary Fig. 7 ), and the electrooxidation temperature (which influences the rate of Cu 2+ and OH – combination, as shown in Supplementary Fig. 8 ). After careful consideration, we decided to use a 2 M aqueous KOH (85%, Wako) electrolyte was used in an ice bath maintained at 0 °C. This setup allowed us to electrochemically oxidize the surface of the cleaned porous Cu foil, leading to the fabrication of needle-like nanostructures with characteristic apex and tilt angles. The electrooxidation process involved maintaining a constant oxidation current density of −4 mA cm −2 for approximately 30 minutes to ensure a high density of needle-like nanostructures. The resulting porous Cu foil was then dried under flowing N 2 for 30 minutes to form porous Cu(OH) 2 . To preserve the original needle-like nanostructure morphology during the reduction of the porous Cu(OH) 2 , we implemented a mild temperature program (3 °C per minute) by gradually heating the porous Cu(OH) 2 to 180 °C over the course of 1 h in an H 2 environment. This step was critical because electrochemical reduction of the porous Cu(OH) 2 would otherwise destroy the original needle-like nanostructure (as illustrated in Supplementary Fig. 9 ). After reaching room temperature, the porous Cu was immersed in an Ar-saturated ethanol solution containing 1-octadecanethiol (10 mM, Wako) at 60 °C for 10 min. This immersion process resulted in the formation of Cu-GDL. Continuous air flushing with Ar was maintained throughout the immersion to ensure the desired result. Characterization X-ray diffraction (XRD) pattern was recorded using a BRUKER D2-Phaser diffractometer at 30 kV and 10 mA using Cu-K α radiation ( λ = 1.54184 Å). Scanning electron microscopy (SEM) images were obtained with a JEOL JSM-7900F microscope. Contact angle measurement was conducted on DM-301 machine. Transmission electron microscope (TEM) images were obtained using a JEOL JEM-ARM200CF microscope operating at 200 kV. X-ray photoemission spectroscopy (XPS) data were collected using an Al-K α radiation source (1486.6 eV) with a PHI 5000 Versa Probe. Attenuation total reflection-Fourier transform infrared (ATR-FTIR) spectra was collected with a Nicolet iS50 spectroscopy. Raman measurement was conducted on an inVia Raman microscope with a 785 nm and 200 µW laser and a 50× objective. Evaluation of electrochemical surface area (ECSA) A 0.1 M KHCO 3 electrolyte saturated with Ar was used for evaluation of electrochemical surface area (ECSA) to determine the electrochemical double-layer capacitance ( C dl ). An electroreduction in potential at −0.6 V versus RHE for 2 min was performed before ECSA evaluation. Cyclic voltammograms were measured at scan rates of 10, 20, 30, 40, and 50 mV·s −1 in the potential range of −0.7 to −0.6 V versus Ag/AgCl. Ar was purged during the measurement. A data set of anodic and cathodic current densities at −0.65 V versus Ag/AgCl was recorded, and the resulting capacitive currents divided by 2 were plotted versus the scan rate. The slope obtained by the linear regression analysis gave the C dl value. Evaluation of surface pH on the electrode All Cu electrodes were reduced at −0.6 V versus RHE for 2 min before cyclic voltammetry (CV) was performed. The CV was conducted in an Ar-saturated 0.1 M KHCO 3 electrolyte at a sweep rate of 10 mV·s −1 while air in the cell was purged with Ar. The surface pH on the electrode was calculated by using following equations: 
    E(vs.RHE)=E(vs.Ag/AgCl)+0.209V+0.0592×pH_surface
 (6) 
    pH_surface=pH_bulk+ΔpH
 (7) where, pH surface is surface pH of the catalyst/electrode, pH bulk is pH of an electrolyte (details in the description of Supplementary Fig. 20 ). In situ Raman spectroscopy measurement A custom-made electrochemical Raman flow cell was used for in situ Raman measurement. A thin electrolyte layer of 5 mm thickness allows the laser to directly irradiate the catalyst surface. A coiled Pt wire (100 × 0.5 mm 2 ) as a counter electrode, and Ag/AgCl (3.0 M NaCl) as a reference electrode were used. Nafion-117 was placed to separate the catholyte and anolyte chambers. The anolyte was 1 M KOH at flow rate of 2.5 mL min −1 , the catholyte was 1 M KCl with pH 6 and pH 1 at a flow rate of 2.5 mL min −1 , and CO 2 was continuously flowed into the gas chamber at a flow rate of 50 mL min −1 during the test. Electrochemical measurements All electrochemical measurements were performed in a gas diffusion flow reactor with a Parstat MC potentiostat (Princeton Applied Research). We used a prepared Cu-GDL as a cathode, a Nafion 117 membrane as a membrane and a Ni foam as an anode, which were positioned and clamped together via gaskets. Unless otherwise stated, a mixed solution of 1 M KCl (99.5%, Wako) and 1 M HCl, and 1 M KOH were used as a catholyte, and circulated through the electrochemical cell using a peristaltic pump with a flow rate of 2.5 ml min −1 , while the CO 2 (99.99%) flow rate was controlled to be 50 ml min −1 . Considering the need for a sustained and stable oxygen evolution reaction to balance the high reaction rate of CO 2 RR, a 1 M KOH was used as the anodic electrolyte. This choice is made due to the use of Nafion 117, a cation exchange membrane, that eliminates OH − crossover to the cathodic side, which affects the pH of the cathodic electrolyte. By using the following equation, the potential versus Ag/AgCl is calibrated in relation to the reversible hydrogen electrode (RHE): E (vs. RHE) = E (vs. Ag/AgCl) + 0.209 V + 0.0592 × pH. The 80% iR drop was compensated by electrochemical impedance spectroscopy (EIS) under open circuit potentials. This EIS test was conducted immediately after each set of CO 2 RR experiments to ensure the accuracy of the internal resistance. Gas chromatography (GC, Agilent 490) was used to analyze effluent gas products extracted from the cathodic compartment, and liquid products were analyzed using high-performance liquid chromatography (HPLC, Shimadzu LC-20AD). Calculations for reaction kinetics The first-order and the second-order reactions are described by following equations; 
    FR_C_2+=k_1 [Cat.] (8) and 
    FR_C_2+=k_2 [Cat.] [OH]
 (9) where \({{{{{\rm{FR}}}}}}_{{{{{{\rm{C}}}}}}_{2+}}\) is formation rate of C 2+ , k 1 and k 2 are the reaction rate constant, [Cat.] and [OH] are the concentration of the catalyst and the OH contained in the catalyst, respectively. Calculations for Faradaic efficiency (FE) and partial current density ( j ) The Faradaic efficiency of gas products (FE gas ) and liquid products (FE liquid ) were calculated based on the following equations: 
    FE_gas=nFC_ivP/QRT× 100%
 (10) 
    FE_liquid=nFC_iV/Q× 100%
 (11) where n is the number of transferred electrons to produce one molecule of the focusing product i , F is the Faraday constant, C i is the concentration of the product i determined by GC or HPLC, v is the flow rate of CO 2 , P , T and Q are pressure, temperature, and total charge followed in the experiment, R is the gas constant, V is the volume of the electrolyte. The partial current density ( j i ) was calculated using: 
    j_i=IFE_i/S
 (12) where I , FE i and S are reaction current, the Faradaic efficiency of the target product i and surface area of the working electrode. Calculation for formation rate (FR), selectivity, single pass conversion efficiency (SPCE) and C 2+ conversion efficiency ( \({{{{{\boldsymbol{CE}}}}}}_{{{{{{\boldsymbol{C}}}}}}_{2+}}\) ) The formation rate, C 2+ selectivity, single pass conversion efficiency and C 2+ conversion efficiency was calculated using: 
    FR_i=QFE_i/nFtS
 (13) 
    Selectivity_i=∑C_i(NFR_i)/∑C_all(NFR_i)× 100%
 (14) 
    SPCE=∑C_all(NFR_i)/v/S× 100%
 (15) 
    CE_C_2+=∑C_2+(NFR_i)/v/S× 100%
 (16) 
    SPCE_i=Selectivity_i×SPCE_t× 100%
 (17) where FR i , Selectivity i , and SPCE i are formation rate, selectivity, single pass conversion efficiency of the target product i , respectively. t and N are reaction time and the number of carbon atoms in each product i , respectively. C all is sum of C i . SPCE t is theoretical maximum SPCE of the target product i when considering the carbonate formation.